Multiple sclerosis-associatedIL2RApolymorphism controls GM-CSF production in human THcells Genome-wide association studies implicate dysregulation of immune mechanisms in the pathogenesis of multiple sclerosis (MS). Particularly, polymorphisms in genes involved in T helper (T H ) cell differentiation are associated with risk of developing MS. However, the underlying mechanism by which these risk alleles influence MS susceptibility has remained elusive. Initiation of neuroinflammation in animal models of MS has been shown to be dependent on T H cell-derived granulocyte-macrophage colony-stimulating factor (GM-CSF). We here report association of GM-CSF expression by human T H cells with MS disease severity. GM-CSF is strongly induced by interleukin 2 (IL-2). We show that an MS-associated polymorphism in the IL-2 receptor alpha ( IL2RA ) gene specifically increases the frequency of GM-CSF-producing T H cells. The IL2RA polymorphism regulates IL-2 responsiveness of naive T H cells and their propensity to develop into GM-CSF-producing memory T H cells. These findings mechanistically link an immunologically relevant genetic risk factor with a functional feature of T H cells in MS. Multiple sclerosis (MS) is a chronic inflammatory disease of the central nervous system with an underlying autoimmune aetiology. The substantially increased risk among relatives and the concordance rate of 30% between identical twins indicate that genetic factors strongly influence the disease susceptibility [1] , [2] . Recent genome-wide association studies demonstrated that single-nucleotide polymorphisms (SNPs) in genes involved in T H cell activation and maturation are over-represented in MS, implicating particularly T H cell differentiation and polarization in MS pathogenesis [3] . Despite the large number of risk factors identified, reports about the underlying molecular mechanisms and their actual contribution to the aetiology of MS remain rare [4] , [5] , [6] . Using animal models of MS, the cytokine granulocyte-macrophage colony-stimulating factor (GM-CSF) was recently identified as the key factor to endow auto-reactive T H cells with the potential to induce neuroinflammation [7] , [8] . Demonstrating its non-redundant function in the initiation and progression of autoimmunity, animals deficient in the GM-CSF ( Csf2 ) gene are resistant to several autoimmune diseases, including experimental autoimmune encephalomyelitis [9] , [10] . GM-CSF regulates the activity of myeloid cells, which form the predominant immune infiltrate in MS brain lesions. Earlier studies showed a correlation between the in vitro administration of interleukin 2 (IL-2) to human T H cells and their secretion of GM-CSF [11] , [12] . IL-2 is a 15-kDa cytokine with pleiotropic functions in promoting T H cell differentiation and effector responses, as well as mediating immune tolerance via regulatory T (T reg ) cells. IL-2 can bind either to its high-affinity receptor, which is composed of three subunits, IL-2Rα (CD25), IL-2Rβ (CD122) and the common γ-chain (γ c or CD132), or to the intermediate affinity receptor consisting of only the IL-2Rβ and γ c [13] . Importantly, IL-2 signalling has been strongly implicated in MS pathogenesis. Attenuation of IL-2 receptor signalling by monoclonal antibodies against the IL-2Rα (daclizumab) reduced the number of gadolinium-enhanced lesions and ameliorated clinical symptoms in a phase II clinical trial in MS patients [14] , [15] . In addition, polymorphisms in the IL2RA are, besides the human leukocyte antigen (HLA) region, the most prominent genetic risk factors of MS [3] , [16] , [17] . The goal of this study was to determine how IL-2R signalling influences T H cell polarization and GM-CSF production in healthy donors versus MS patients, and whether modulation of T H cell differentiation by IL2RA polymorphisms is associated with increased risk of developing MS. Using a large cohort of patients, we found the frequency of GM-CSF-producing T H cells to be significantly increased in MS patients versus patients suffering from other non-inflammatory neurological diseases (OND). Also, GM-CSF + T H cell frequencies are associated with biomarkers of disease severity and are decreased upon immunomodulatory therapy. Among the cytokines tested, IL-2 engagement of its trimeric receptor complex and signalling through the signal transducer and activator of transcription 5 (STAT5) was the strongest inducer of GM-CSF in human T H cells in vitro . We found that MS-associated polymorphisms in the IL2RA , but not other risk alleles tested, increased the frequency of GM-CSF-producing T H cells in healthy individuals. The data presented provide a molecular connection between a major genetic risk factor of MS and its impact on the formation of potentially pathogenic T H cells in humans. IL-2 induces the production of GM-CSF in human T H cells To reveal the most potent inducer of GM-CSF production in human T H cells, we activated (αCD3/αCD28, irradiated feeder cells) naive T H cells from healthy donors in the presence of IL-23, IL-1β and IL-6, which have been demonstrated to drive GM-CSF secretion in murine T H cells [7] , [8] or with IL-2. IL-23, IL-1β and IL-6 did not increase GM-CSF production by human T H cells ( Fig. 1a,b ). Importantly, we noticed that IL-2 was able to substantially increase the expression of GM-CSF by human T H cells. Moreover, GM-CSF production observed without addition of exogenous cytokines was dependent on endogenously produced IL-2 ( Fig. 1c ). Addition of transforming growth factor (TGF)-β1 or TGF-β3 to induce IL-17A production negatively regulated GM-CSF secretion ( Fig. 1a,b,d–f ), similar to what has been observed in murine T cells [8] . The frequency of IL-2Rα + T H cells was not affected by TGF-β ( Fig. 1f–h ). 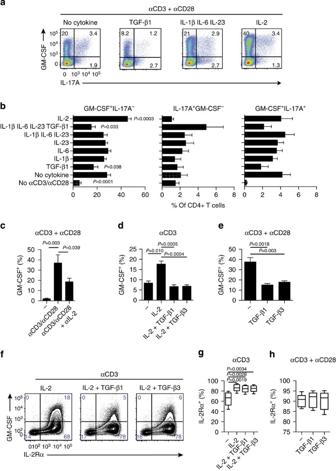Figure 1: IL-2 drives GM-CSF secretion by human THcells. (a) Representative and (b) cumulative frequencies of sorted naive THcells (CD4+CD45RO−CD62L+), activated (αCD3/αCD28) in the presence of 10 ng ml−1of the indicated cytokines. The frequency of GM-CSF+IL-17A−, IL-17A+GM-CSF−and GM-CSF+IL-17A+was determined by flow cytometry on day 7 (n=6). Data are combined from >3 independent experiments. (c) Naive THcells were activated (αCD3/αCD28) in the presence or absence of neutralizing IL-2 antibody (n=7). Data are combined from three independent experiments. (d–h) Naive THcells were activated as indicated in the presence or absence of the indicated TGF-β for 5 days (n=5). Shown are cumulative results of GM-CSF+THcells after αCD3 activation (d) or after αCD3/ αCD28 activation (e), representative flow cytometric results (f) and cumulative results of IL-2Rα expression on THcells after αCD3 activation (g) and after αCD3/ αCD28 activation (h). For all figures error bars show mean±s.e.m. Figure 1: IL-2 drives GM-CSF secretion by human T H cells. ( a ) Representative and ( b ) cumulative frequencies of sorted naive T H cells (CD4 + CD45RO − CD62L + ), activated (αCD3/αCD28) in the presence of 10 ng ml −1 of the indicated cytokines. The frequency of GM-CSF + IL-17A − , IL-17A + GM-CSF − and GM-CSF + IL-17A + was determined by flow cytometry on day 7 ( n =6). Data are combined from >3 independent experiments. ( c ) Naive T H cells were activated (αCD3/αCD28) in the presence or absence of neutralizing IL-2 antibody ( n =7). Data are combined from three independent experiments. ( d – h ) Naive T H cells were activated as indicated in the presence or absence of the indicated TGF-β for 5 days ( n =5). Shown are cumulative results of GM-CSF + T H cells after αCD3 activation ( d ) or after αCD3/ αCD28 activation ( e ), representative flow cytometric results ( f ) and cumulative results of IL-2Rα expression on T H cells after αCD3 activation ( g ) and after αCD3/ αCD28 activation ( h ). For all figures error bars show mean±s.e.m. Full size image IL-2Rα engagement drives GM-CSF in human T H cells CD28 costimulation is a strong inducer of IL-2 production in T cells. To precisely control IL-2 levels, we activated naive T H cells with only αCD3 in the presence of irradiated feeder cells and the respective cytokines. Addition of IL-6 and IL-1β led to a moderate increase in the frequency of GM-CSF-producing T H cells, but only marginally affected the concentration of secreted GM-CSF ( Fig. 2a,b ). In contrast, IL-2 induced a strong increase in the frequency, as well as in the level of secreted GM-CSF. IL-2 promoted GM-CSF in a dose-dependent manner, in terms of the frequency of cytokine-producing T H cells, as well as in the level of secreted cytokine ( Fig. 2c,d ). Production of other cytokines such as interferon (IFN)-γ was only mildly increased. Similar to the frequency of GM-CSF-secreting cells, IL-2Rα + T H cells increased depending on the IL-2 concentration ( Fig. 2e ). Of note, the employed concentrations of recombinant IL-2 were within the range of IL-2 levels measured in the serum of healthy individuals ( Fig. 2f ). After activation in the presence of IL-2, all GM-CSF-producing T H cells expressed the IL-2Rα ( Fig. 2g,h ). This expression was critical for the induction of GM-CSF through IL-2, as shown by blocking of IL-2Rα with monoclonal antibodies, which drastically reduced GM-CSF secretion by T H cells ( Fig. 2i ). Together, this highlights the importance of the IL-2Rα for the induction of GM-CSF production by human T H cells. 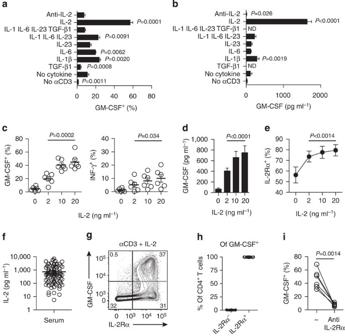Figure 2: IL-2Rα is critical for the induction of GM-CSF. (a,b) Sorted naive THcells (CD4+CD45RO−CD25−/medCD127+) were activated (αCD3) in the presence of 10 ng ml−1of the indicated cytokine for 5 days (n=6). Shown are cumulative results of GM-CSF+in THcells (a) and the level of secreted GM-CSF in the cell culture supernatant (b). ND, not detected. (c–e) Naive THcells as inaandbwere activated (αCD3) in the presence of the indicated concentration of IL-2 for 5 days. Shown are the frequency of GM-CSF+and IFN-γ+THcells (c,n=6), GM-CSF levels in the cell culture supernatant (d,n=12) and the frequency of IL-2Rα+THcells (e,n=4). (f) GM-CSF levels in serum of healthy individuals was analysed by the enzyme-linked immunosorbent assay (n=99). Data are combined from three independent experiments. (g,h) Representative example (g) and cumulative results (h) of sorted naive THcells, which were activated (αCD3) in the presence of 10 ng ml−1IL-2 and analysed for GM-CSF secretion and IL-2Rα expression on day 5 (n=12). Data are combined from three independent experiments. (i) Blocking of the IL-2Rα by monoclonal antibodies during the activation of naive THcells in the presence of 10 ng ml−1IL-2 for 5 days (n=6). Data are combined from three independent experiments. For all figures error bars show mean±s.e.m. Figure 2: IL-2Rα is critical for the induction of GM-CSF. ( a , b ) Sorted naive T H cells (CD4 + CD45RO − CD25 −/med CD127 + ) were activated (αCD3) in the presence of 10 ng ml −1 of the indicated cytokine for 5 days ( n =6). Shown are cumulative results of GM-CSF + in T H cells ( a ) and the level of secreted GM-CSF in the cell culture supernatant ( b ). ND, not detected. ( c – e ) Naive T H cells as in a and b were activated (αCD3) in the presence of the indicated concentration of IL-2 for 5 days. Shown are the frequency of GM-CSF + and IFN-γ + T H cells ( c , n =6), GM-CSF levels in the cell culture supernatant ( d , n =12) and the frequency of IL-2Rα + T H cells ( e , n =4). ( f ) GM-CSF levels in serum of healthy individuals was analysed by the enzyme-linked immunosorbent assay ( n =99). Data are combined from three independent experiments. ( g , h ) Representative example ( g ) and cumulative results ( h ) of sorted naive T H cells, which were activated (αCD3) in the presence of 10 ng ml −1 IL-2 and analysed for GM-CSF secretion and IL-2Rα expression on day 5 ( n =12). Data are combined from three independent experiments. ( i ) Blocking of the IL-2Rα by monoclonal antibodies during the activation of naive T H cells in the presence of 10 ng ml −1 IL-2 for 5 days ( n =6). Data are combined from three independent experiments. For all figures error bars show mean±s.e.m. Full size image IL-2 drives GM-CSF production independent of proliferation IL-2 is known to drive T H cell expansion. We therefore tested whether this might contribute to the observed increase in the frequency of GM-CSF-secreting T H cells. We activated naive T H cells in the presence of IL-2, IL-7 or IL-15, cytokines known to promote T H cell expansion ( Fig. 3a ). IL-2 and IL-15 both induced strong GM-CSF production in T H cells ( Fig. 3a,b ). IL-7 strongly stimulated proliferation while it only slightly affected the frequency of GM-CSF-secreting T H cells, indicating that expansion per se is not sufficient to induce GM-CSF production ( Fig. 3a,b ). Consequently, the frequency of GM-CSF-secreting T H cells did not correlate with the calculated percentage of divided cells ( Fig. 3c ). To further support this, we determined the cell-cycle state of GM-CSF-secreting cells after activation of T H cells in the presence of those cytokines. IL-2, IL-7 and IL-15 all induced proliferation ( Fig. 3d ), however, we found that the majority of GM-CSF-secreting cells were not actively proliferating, thus demonstrating that proliferation is not essential for GM-CSF production ( Fig. 3e,f ). 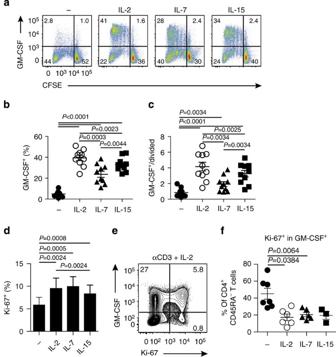Figure 3: GM-CSF secretion is independent of proliferation. (a) Representative examples and (b) cumulative results of sorted naive THcells that were activated (αCD3) in the presence of 10 ng ml−1of IL-2, IL-7 or IL-15 and analysed for GM-CSF expression and proliferation (carboxyfluorescein succinimidyl ester (CFSE)-dilution) on day 5 (n=10). (c) Normalization of the frequency of GM-CSF-secreting THcells by the calculated frequency of divided THcells (n=10). Data are combined from >3 independent experiments. (d,e) Cumulative results (d) and representative example (e) of purified THcells that were activated (αCD3) in the presence of the indicated cytokines and analysed for cell-cycle state and GM-CSF production on day 2 (n=8). (f) Frequency of proliferating (Ki-67+) THcells within the fraction of GM-CSF+THcells after activation in the presence of 10 ng ml−1of the indicated cytokine for 4 days (n=7,6,6,3, respectively). Data are from one representative of two independent experiments. Each symbol represents a single individual. For all figures error bars show mean±s.e.m. Figure 3: GM-CSF secretion is independent of proliferation. ( a ) Representative examples and ( b ) cumulative results of sorted naive T H cells that were activated (αCD3) in the presence of 10 ng ml −1 of IL-2, IL-7 or IL-15 and analysed for GM-CSF expression and proliferation (carboxyfluorescein succinimidyl ester (CFSE)-dilution) on day 5 ( n =10). ( c ) Normalization of the frequency of GM-CSF-secreting T H cells by the calculated frequency of divided T H cells ( n =10). Data are combined from >3 independent experiments. ( d , e ) Cumulative results ( d ) and representative example ( e ) of purified T H cells that were activated (αCD3) in the presence of the indicated cytokines and analysed for cell-cycle state and GM-CSF production on day 2 ( n =8). ( f ) Frequency of proliferating (Ki-67 + ) T H cells within the fraction of GM-CSF + T H cells after activation in the presence of 10 ng ml −1 of the indicated cytokine for 4 days ( n =7,6,6,3, respectively). Data are from one representative of two independent experiments. Each symbol represents a single individual. For all figures error bars show mean±s.e.m. Full size image GM-CSF expression is regulated via STAT5 IL-2 and IL-15 both induce strong phosphorylation of STAT5. We investigated whether this signalling pathway is initiating GM-CSF induction in human T H cells. Therefore, we stimulated T H cells with different γ c -cytokines or different IL-2 concentrations to induce varying levels of pSTAT5. The frequency of GM-CSF + T H cells closely correlated with STAT5 phosphorylation, indicating that pSTAT5 directly drives GM-CSF expression ( Fig. 4a,b ). Using in silico analysis, we found the human GM-CSF ( CSF2 ) promoter to contain a STAT5-binding site (chr5:131,409,289–131,409,300). Further supporting this concept, we observed loss of IL-2-induced GM-CSF production on protein and messenger RNA levels upon specific STAT5 inhibition [18] in T H cells ( Fig. 4c–e ). GM-CSF production induced by endogenous IL-2 was similarly reduced by STAT5 inhibition. 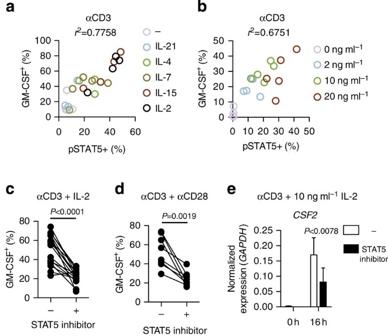Figure 4: IL-2 induces GM-CSF via phosphorylation of STAT5. (a,b) Sorted naive THcells (CD4+CD45RO−CD25−/medCD127+) were activated (αCD3) in the presence of the indicated cytokine for 5 days. GM-CSF secretion and STAT5 phosphorylation (10 min of restimulation with the indicated cytokine in the same concentration) were analysed by flow cytometry on day 5. Shown are the frequencies of GM-CSF+versus pSTAT5+THcells after stimulation in the presence of different γc-cytokines (a,n=4) and after stimulation with different IL-2 concentrations (b,n=5). Data are from one representative of two independent experiments. (c,d) Naive THcells as inaandbwere activated with αCD3+IL-2 (c,n=16) or αCD3/αCD28 (d,n=8) with or without inhibition of STAT5 phosphorylation (2.5 μg ml−1pimozide). Data are combined from two independent experiments. (e) Purified THcells were activated (αCD3) in the presence of IL-2 with or without the STAT5 inhibitor for 16 h beforeCSF2messenger RNA levels were analysed by quantitative real-time PCR (n=8). Data are combined from two independent experiments. Each symbol represents a single individual. For all figures error bars show mean±s.e.m. Figure 4: IL-2 induces GM-CSF via phosphorylation of STAT5. ( a , b ) Sorted naive T H cells (CD4 + CD45RO − CD25 −/med CD127 + ) were activated (αCD3) in the presence of the indicated cytokine for 5 days. GM-CSF secretion and STAT5 phosphorylation (10 min of restimulation with the indicated cytokine in the same concentration) were analysed by flow cytometry on day 5. Shown are the frequencies of GM-CSF + versus pSTAT5 + T H cells after stimulation in the presence of different γc-cytokines ( a , n =4) and after stimulation with different IL-2 concentrations ( b , n =5). Data are from one representative of two independent experiments. ( c , d ) Naive T H cells as in a and b were activated with αCD3+IL-2 ( c , n =16) or αCD3/αCD28 ( d , n =8) with or without inhibition of STAT5 phosphorylation (2.5 μg ml −1 pimozide). Data are combined from two independent experiments. ( e ) Purified T H cells were activated (αCD3) in the presence of IL-2 with or without the STAT5 inhibitor for 16 h before CSF2 messenger RNA levels were analysed by quantitative real-time PCR ( n =8). Data are combined from two independent experiments. Each symbol represents a single individual. For all figures error bars show mean±s.e.m. Full size image T reg cells inhibit GM-CSF + T H cells through IL-2 deprivation T reg cells are capable of regulating cytokine secretion by auto-aggressive T cells through various mechanisms (reviewed in ref. 19 ), and alterations in this suppression have been reported in MS patients [20] , [21] . We found T reg cells to suppress IL-2-induced STAT5 phosphorylation (data not shown) and subsequent GM-CSF production by conventional T H cells ( Fig. 5a,b ). This suppression functions mostly independently of TGF-β or IL-10, but rather through deprivation of IL-2 ( Fig. 5c ). Regulation of IL-2 levels by T reg cells thus has a major impact on the effector function of T H cells through direct modulation of GM-CSF production. 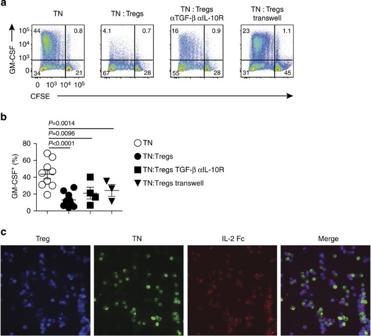Figure 5: Regulatory T cells suppress GM-CSF production by deprivation of IL-2. (a,b) Sorted naive (TN) and regulatory T cells (Treg) were co-cultured in a 1:1 ratio and activated (αCD3/αCD28) and the indicated blocking antibodies for 5 d (n=9,9,4,3, respectively). Shown are representative examples of GM-CSF secretion and carboxyfluorescein succinimidyl ester (CFSE) dilution (a) and cumulative results of GM-CSF secretion (b). Data are combined from three independent experiments. (c) Fluorescent imaging of TN(CFSE labelled) and Tregcells (CellTrace Violet labelled), which were stimulated together with 10 ng ml−1IL-2Fc for 10 min. Each symbol represents a single individual. For all figures error bars show mean±s.e.m. Figure 5: Regulatory T cells suppress GM-CSF production by deprivation of IL-2. ( a , b ) Sorted naive (T N ) and regulatory T cells (T reg ) were co-cultured in a 1:1 ratio and activated (αCD3/αCD28) and the indicated blocking antibodies for 5 d ( n =9,9,4,3, respectively). Shown are representative examples of GM-CSF secretion and carboxyfluorescein succinimidyl ester (CFSE) dilution ( a ) and cumulative results of GM-CSF secretion ( b ). Data are combined from three independent experiments. ( c ) Fluorescent imaging of T N (CFSE labelled) and T reg cells (CellTrace Violet labelled), which were stimulated together with 10 ng ml −1 IL-2Fc for 10 min. Each symbol represents a single individual. For all figures error bars show mean±s.e.m. Full size image GM-CSF-secreting T H cells are elevated in MS patients GM-CSF is currently considered to be a promising therapeutic target in several autoimmune diseases, such as rheumatoid arthritis [22] and MS (NCT01517282). Therefore, we quantified the ex vivo frequency of GM-CSF-, IL-17A- and IFN-γ-secreting memory T H cells in the peripheral blood of MS patients compared with OND patients ( Supplementary Tables 1–3 ). We observed that untreated MS patients had a significantly higher frequency of GM-CSF-producing memory T H cells compared with OND patients (17.0% versus 11.5%, Fig. 6a,b ). A similar 1.5-fold increase (15.5% versus 10.1%) was observed in an independent validation cohort of MS and OND patients, yet marginally above the statistical threshold ( P =0.052, Supplementary Fig. 1a ). In addition, we could replicate the previously reported [23] increase in IFN-γ-producing memory T H cells in MS versus OND (21.7% versus 16.0%). In agreement with previous reports [24] , we observed only a modest increase (1.0% versus 0.8%) in the frequency of IL-17A-secreting T H cells. Interestingly, patients treated with immunemodulatory drugs had a significantly reduced frequency of GM-CSF-secreting T H cells compared with untreated patients (10.8% versus 17.0%, Fig. 6a,c ; Supplementary Fig. 1b ). A similar effect of immunomodulatory treatment, albeit less pronounced, was observed in the frequency of IFN-γ-producing memory T H cells (17.3% versus 21.7%). We did not observe any significant difference in the percentage of IL-17A-producing memory T H cells upon therapy. The proportion of IL-2Rα + memory T H cells did not significantly differ between the patient groups ( Supplementary Fig. 1c ). Taken together, GM-CSF + T H cell frequencies are elevated in MS and decrease upon immunemodulatory therapy. 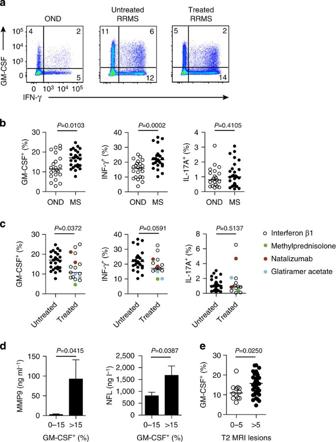Figure 6: MS patients have elevated frequencies of GM-CSF-secreting THmemory cells. (a) Representative GM-CSF and IFN-γ production and (b) cumulative data from PBMCs of untreated relapsing-remitting MS (RRMS) patients and OND patients, which were analysedex vivo(no previousin vitroculture) for the frequency of total GM-CSF+, IFN-γ+and IL-17A+memory THcells by flow cytometry (ONDn=22; MSn=27). (c) Effect of immunemodulatory treatment on theex vivofrequency of peripheral GM-CSF+, IFN-γ+(untreatedn=27, treatedn=17) and IL-17A+(untreatedn=27, treatedn=16) memory THcells. Data are combined from >3 independent experiments. (d) CSF serum levels of MMP9 and NFL in RRMS patients with a low (n=14) or high (n=14) frequency of GM-CSF+memory THcells. (e)Ex vivofrequency of GM-CSF+memory THcells in MS patients (RRMS/CIS) with 0–5 (n=12) versus MS patients with >5 (n=39) T2 magnetic resonance imaging (MRI) lesions. Data are combined from >3 independent experiments. Each circle represents a single individual. (b,c,e) Lines represent the median, (d) error bars show mean±s.e.m. Figure 6: MS patients have elevated frequencies of GM-CSF-secreting T H memory cells. ( a ) Representative GM-CSF and IFN-γ production and ( b ) cumulative data from PBMCs of untreated relapsing-remitting MS (RRMS) patients and OND patients, which were analysed ex vivo (no previous in vitro culture) for the frequency of total GM-CSF + , IFN-γ + and IL-17A + memory T H cells by flow cytometry (OND n =22; MS n =27). ( c ) Effect of immunemodulatory treatment on the ex vivo frequency of peripheral GM-CSF + , IFN-γ + (untreated n =27, treated n =17) and IL-17A + (untreated n =27, treated n =16) memory T H cells. Data are combined from >3 independent experiments. ( d ) CSF serum levels of MMP9 and NFL in RRMS patients with a low ( n =14) or high ( n =14) frequency of GM-CSF + memory T H cells. ( e ) Ex vivo frequency of GM-CSF + memory T H cells in MS patients (RRMS/CIS) with 0–5 ( n =12) versus MS patients with >5 ( n =39) T2 magnetic resonance imaging (MRI) lesions. Data are combined from >3 independent experiments. Each circle represents a single individual. ( b , c , e ) Lines represent the median, ( d ) error bars show mean±s.e.m. Full size image GM-CSF + T H cells coincide with biomarkers for MS severity Furthermore, we analysed whether increased GM-CSF production by T H cells is associated with cerebrospinal fluid (CSF) biomarkers of disease progression and severity such as matrix metalloproteinase 9 (MMP9), an indicator of brain–blood barrier integrity [25] , as well as neurofilament-light chain (NFL), a marker for neuronal damage [26] . MS patients with an elevated frequency (above a median of 15.3%) of GM-CSF-secreting T H cells had strongly elevated CSF levels of MMP9 (2.9 versus 92.4 ng ml −1 , Fig. 6d ) as well as NFL (810 versus 1677, ng l −1 ), compared with MS patients with a low (below median) frequency of GM-CSF-producing T H cells. In addition, we observed an increase in GM-CSF-producing T H cells in MS patients with more T2 magnetic resonance imaging lesions ( Fig. 6e ). Taken together, these observations indicate that patients with higher proportions of GM-CSF-producing T H cells may have a more severe MS phenotype. IL2RA risk alleles increase the frequency of GM-CSF + T H cells Given the relationship between MS and the frequency of GM-CSF + -producing T H cells, together with the role of IL-2 in the regulation of GM-CSF, we tested whether MS-associated IL2RA polymorphisms modulate GM-CSF production and thereby increase the risk of MS in healthy individuals (see Supplementary Table 4 ). In agreement with previous reports [27] , we observed increased surface expression of IL-2Rα on naive T H cells in individuals with rs2104286 risk (A/A) versus protective alleles (A/G or G/G, see Supplementary Table 5 ; Fig. 7a ). We analysed whether this risk allele-mediated increase in IL-2 responsiveness of naive T H cells translates into corresponding frequencies of GM-CSF-producing memory T H cells. In vitro stimulation (αCD3 and 10 ng ml −1 IL-2) of sorted naive T H cells with rs2104286 risk alleles resulted in higher frequencies of GM-CSF-producing memory T H cells when compared with T H cells carrying protective alleles ( Fig. 7b ). In addition, sorted IL-2Rα + naive T H cells produced higher levels of GM-CSF after activation, in the presence of IL-2 compared with their IL-2Rα − counterpart ( Fig. 7c ). We next analysed whether this modulation of GM-CSF production also occurs in vivo , and observed that individuals with rs2104286 risk alleles had a substantially increased number of GM-CSF-producing memory T H cells compared with individuals with protective alleles ( Fig. 7d ). The frequency of IFN-γ- and IL-17A-secreting memory T H cells was not affected by rs2104286. 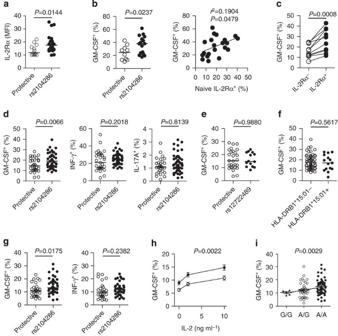Figure 7: MS-associatedIL2RArisk alleles augment GM-CSF-producing THcells. (a)Ex vivosurface expression of IL-2Rα on naive THcells from healthy individuals with a protective (G/G or A/G) or riskIL2RAgenotype (A/A) at rs2104286, determined by flow cytometry (protectiven=14, rs2104286n=25). Data are combined from >3 independent experiments. (b) Sorted naive THcells were activatedin vitro(αCD3) in the presence of 10 ng ml−1IL-2 and then analysed for GM-CSF expression by flow cytometry on day 5 (protectiven=10, rs2104286n=16). Data are combined from >3 independent experiments. (c) Naive THcells were sorted according to IL-2Rα expression and then activated (αCD3) for 5 days in the presence of 10 ng ml−1IL-2 (n=10). Data are combined from two independent experiments. (d) PBMCs from healthy individuals were analysedex vivo(without previousin vitroculture) for the frequency of GM-CSF+, IFN-γ+and IL-17A+memory THcells (protectiven=31, rs2104286n=46). (e) Individuals with rs2104286 protective alleles were further analysed forex vivoGM-CSF expression with regard to rs12722489 (protectiven=28, rs12722489n=14). (f)Ex vivofrequency of GM-CSF+THcells with regard to HLA-DRB1*15:01 alleles (HLA-DRB1*15:01−n=58, HLA-DRB1*15:01+n=15). Data are combined from >3 independent experiments. (g,h) Purified THcells were cultured in the presence of 0–10 ng ml−1IL-2 (no αCD3) for 4 days. Shown are the frequency of GM-CSF+and IFN-γ+THcells at 10 ng ml−1IL-2 (protectiven=28, rs2104286n=40,g) and the frequency of GM-CSF+THcells at IL-2 concentrations from 0 to 10 ng ml−1(protectiven=30, rs2104286n=34,h). (i) Gene-dosage effect of rs2104286 on the frequency of GM-CSF+THcells, cultured as ingandh, assuming a linear gene–phenotype relation (G/Gn=5, A/Gn=33, A/An=45). Data are combined from >3 independent experiments. Each symbol represents a single individual. (a–g) lines represent the median, (h,i) error bars show mean±s.e.m. Figure 7: MS-associated IL2RA risk alleles augment GM-CSF-producing T H cells. ( a ) Ex vivo surface expression of IL-2Rα on naive T H cells from healthy individuals with a protective (G/G or A/G) or risk IL2RA genotype (A/A) at rs2104286, determined by flow cytometry (protective n =14, rs2104286 n =25). Data are combined from >3 independent experiments. ( b ) Sorted naive T H cells were activated in vitro (αCD3) in the presence of 10 ng ml −1 IL-2 and then analysed for GM-CSF expression by flow cytometry on day 5 (protective n =10, rs2104286 n =16). Data are combined from >3 independent experiments. ( c ) Naive T H cells were sorted according to IL-2Rα expression and then activated (αCD3) for 5 days in the presence of 10 ng ml −1 IL-2 ( n =10). Data are combined from two independent experiments. ( d ) PBMCs from healthy individuals were analysed ex vivo (without previous in vitro culture) for the frequency of GM-CSF + , IFN-γ + and IL-17A + memory T H cells (protective n =31, rs2104286 n =46). ( e ) Individuals with rs2104286 protective alleles were further analysed for ex vivo GM-CSF expression with regard to rs12722489 (protective n =28, rs12722489 n =14). ( f ) Ex vivo frequency of GM-CSF + T H cells with regard to HLA-DRB1*15:01 alleles (HLA-DRB1*15:01 − n =58, HLA-DRB1*15:01 + n =15). Data are combined from >3 independent experiments. ( g , h ) Purified T H cells were cultured in the presence of 0–10 ng ml −1 IL-2 (no αCD3) for 4 days. Shown are the frequency of GM-CSF + and IFN-γ + T H cells at 10 ng ml −1 IL-2 (protective n= 28, rs2104286 n =40, g ) and the frequency of GM-CSF + T H cells at IL-2 concentrations from 0 to 10 ng ml −1 (protective n =30, rs2104286 n= 34, h ). ( i ) Gene-dosage effect of rs2104286 on the frequency of GM-CSF + T H cells, cultured as in g and h , assuming a linear gene–phenotype relation (G/G n =5, A/G n =33, A/A n =45). Data are combined from >3 independent experiments. Each symbol represents a single individual. ( a – g ) lines represent the median, ( h , i ) error bars show mean±s.e.m. Full size image Several SNPs have been identified within the IL2RA locus, including rs12722489, which is in modest linkage disequilibrium with rs2104286. Recent data show that of these two, only rs2104286 increases the risk to develop MS [17] . Accordingly, rs12722489 did not alter the frequency of GM-CSF-producing T H cells, demonstrating that the observed increase in GM-CSF production by rs2104286 is a specific consequence of risk-driving genetic variants and not other IL2RA SNPs ( Fig. 7e ). Furthermore, we found the strongest genetic association with MS, HLA-DRB1*15:01, to have no influence on the frequency of GM-CSF-expressing T H cells ( Fig. 7f ), indicating that modulation of GM-CSF expression is not a general mechanism of MS-associated risk genes. In addition, HLA-DRB1*15:01 has been reported to enhance autologous T-cell proliferation [28] , further indicating that elevated proliferation is largely disconnected from the observed increase in GM-CSF production. IL2RA influence on GM-CSF is preserved upon IL-2R engagement To directly assess the impact of the IL2RA SNP rs2104286 on IL-2R signalling, we additionally measured GM-CSF secretion after stimulating T H cells with IL-2 in the absence of TCR-engagement. Individuals with MS-associated risk alleles again showed a significantly higher number of GM-CSF-secreting T H cells compared with donors carrying protective alleles ( Fig. 7g ). As observed also immediately ex vivo , the frequency of IFN-γ-secreting T H cells did not differ significantly between groups upon IL-2 stimulation. The increased frequency of GM-CSF-producing T H cells in individuals with rs2104286 risk alleles was maintained at different IL-2 concentrations ( Fig. 7h ). Finally, we observed a gene-dosage effect of the MS-associated rs2104286 risk allele on the frequency of IL-2-stimulated GM-CSF-secreting T H cells ( Fig. 7i ). We found that GM-CSF production by CD8 + T cells is not modulated by MS-associated risk genes or by MS disease ( Fig. 8a–c ). This specificity therefore underlines the importance of GM-CSF production by human T H cells in the context of MS pathology. 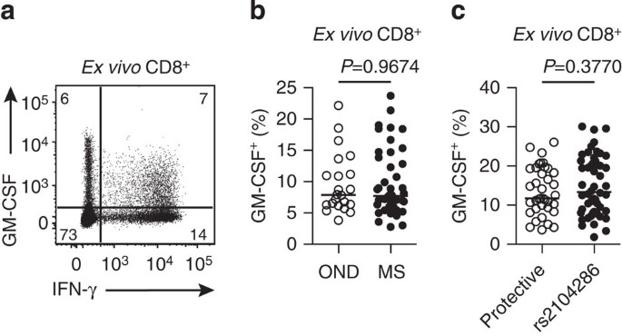Figure 8: GM-CSF production by CD8+T cells is not altered in the context of MS. (a–c) The frequency of cytokine-secreting CD8+T cells determined by flow cytometry without priorin vitroculture. Shown are a representative GM-CSF and IFN-γ secretion profile of CD8+T cells (a), cumulative frequencies of GM-CSF-secreting CD8+T cells from untreated MS (n=27) versus OND patients (n=22;b) and cumulative frequencies of GM-CSF-secreting CD8+T cells with a protective (G/G or A/G) or riskIL2RAgenotype (A/A) at rs2104286 (protectiven=37, rs2104286n=52;c). Data are combined from >3 independent experiments. Each circle represents a single individual. Throughout all figures lines represent the median. Figure 8: GM-CSF production by CD8 + T cells is not altered in the context of MS. ( a – c ) The frequency of cytokine-secreting CD8 + T cells determined by flow cytometry without prior in vitro culture. Shown are a representative GM-CSF and IFN-γ secretion profile of CD8 + T cells ( a ), cumulative frequencies of GM-CSF-secreting CD8 + T cells from untreated MS ( n =27) versus OND patients ( n =22; b ) and cumulative frequencies of GM-CSF-secreting CD8 + T cells with a protective (G/G or A/G) or risk IL2RA genotype (A/A) at rs2104286 (protective n =37, rs2104286 n =52; c ). Data are combined from >3 independent experiments. Each circle represents a single individual. Throughout all figures lines represent the median. Full size image The molecular signature and functional properties of auto-aggressive T cells in chronic inflammatory disease remain a subject of intense research [29] . GM-CSF emerges as a major pro-inflammatory mediator in preclinical models of autoimmune disease. For instance, T cells deficient in GM-CSF fail to transfer disease in an animal model of MS. Thus GM-CSF has, in contrast to IL-17A or IFN-γ, a non-redundant function in the development of autoimmune neuroinflammation [7] . Of note, a recent phase II clinical trial showed therapeutic efficacy of GM-CSF neutralization in rheumatoid arthritis patients [30] (NCT01023256); GM-CSF neutralization trials are also currently ongoing in MS patients (NCT01517282). Supporting the involvement of GM-CSF in MS, we here report increased frequencies of GM-CSF-producing T H cells in MS compared with control patients. In addition, we found increased levels of CSF biomarkers of MS disease progression and severity, as well as the number of magnetic resonance imaging lesions, to correspond with GM-CSF expression in these patients. Interestingly, immunomodulatory therapy in MS coincided with a reduction in the frequency of GM-CSF (but not IL-17A or IFN-γ)-secreting T cells. This is not likely due to a direct impact of therapeutic interventions on GM-CSF production, but rather that therapy-induced reduction in disease activity leads to a normalization of GM-CSF frequencies in T H cells. In contrast to mice, where numerous cytokines have been proposed to initiate GM-CSF transcription [8] , we observed that in humans, IL-2 is a particularly strong driver of GM-CSF production. In agreement with others, we found the GM-CSF-inducing capacity of IL-2 to be independent of the effect IL-2 has on proliferation [31] . Genome-wide association studies firmly link polymorphisms in the IL2RA locus with the risk to develop MS. However, the mechanism by which the IL2RA polymorphism rs2104286 confers this risk has been elusive. Here we found a significantly increased propensity of T H cells from individuals carrying IL2RA risk alleles to secrete GM-CSF. Rs2104286 is an intronic SNP, which has been shown to regulate messenger RNA expression of IL-2Rα [27] . We here confirm that individuals with rs2104286 risk alleles have increased levels of surface IL-2Rα on naive T H cells. This elevated responsiveness of naive T H cells from healthy individuals with risk alleles results in a higher propensity to develop GM-CSF-expressing effector T H cells. This finding mechanistically links a prominent genetic risk factor with the production of the pro-inflammatory cytokine GM-CSF by T H cells, extending previous studies exploring possible pathogenic mechanisms of IL2RA SNPs [27] , [32] , [33] , [34] . Taken together, our study resolves and integrates findings obtained in preclinical models with human disease by providing a direct link between a genetic risk trait in MS pathogenesis, IL-2R signalling and a feature of pathogenic T cells, namely GM-CSF production. Healthy donor and patient samples Blood samples from healthy volunteers ( Supplementary Table 3 ) were recruited via the blood donation centre, Zurich, Switzerland with approval of the cantonal ethics committee, Zurich. MS and OND patient samples (see Supplementary Tables 1 and 2 ) were collected at the neurological clinics at Karolinska University Hospitals Solna and Huddinge. MS and OND samples for validation were collected at the Nottingham University Hospitals, UK. Informed consent was collected from all participants. DNA was isolated using the DNeasy blood and tissue kit (Qiagen). SNPs and the HLA-DRB1*15:01 (rs3135388 (refs 16 , 35 )) genotype were determined using TaqMan SNP Genotyping Assays (Life technologies). Flow cytometric experiments and analysis was performed blinded with regard to disease and genotype. Flow cytometry and cell sorting To sort naive T H cells (CD4 + CD127 + CD25 −/med CD45RO − ) from healthy donors, total peripheral blood mononucleated cells (PBMCs) were stained with anti-human CD4 APC-Cy7 (RPA-T4, 1/100, BD Pharmingen), CD25 APC (BC96, 1/50, eBioscience), CD127 FITC (eBioRDR5, 1/50, eBioscience) and CD45RO ECD (HI100, 1/100, Beckman Coulter). T reg cells were defined as CD4 + CD127 − CD25 high and excluded from the naive T H cell population. Anti-human monoclonal antibodies used for ex vivo surface staining were PacificBlue-conjugated CD4 (RPA-T4, 1/200, Biolegend), Brilliant Violet 785-conjugated CD8 (RPA-T8, 1/200, Biolegend), APC-conjugated CD25 (BC96, 1/50, eBiosciences) and PE-Cy7-conjugated CD45RA (HI100, 1/200, Biolegend). Intracellular cytokine staining was performed using anti-human PE-conjugated GM-CSF (BVD2-21C11, 1/200, BD Biosciences), Alexa Fluor 488-conjugated or PE-Cy7-conjugated IFN-γ (4S.B3, both 1/200, Biolegend or eBiosciences), APC-Cy7-conjugated IL-17A (BL168, 1/200, Biolegend) and AlexaFluor 488-conjugated IL-4 (8D4–8, 1/50, Biolegend). Dead cells were excluded using the LIVE/DEAD fixable dead cell stain kit (Invitrogen). The frequency of cytokine-secreting cells was determined after short restimulation using 50 ng ml −1 phorbol 12-myristate 13-acetate (PMA) and 500 ng ml −1 ionomycin in the presence of a protein transport inhibitor (Golgiplug, BD) for 4 h before fixation and intracellular staining. For STAT5 phosphorylation assays, anti-human APC-conjugated CD4 (RPA-T4, 1/20, Biolegend) and PE or APC-conjugated pSTAT5 (47, both 1/20, BD Biosciences and C71E5, Cell signaling technology, respectively) were used. Cell cycle analysis was performed using FITC-conjugated anti-human Ki-67 (35/Ki-67, 1/20, BD Biosciences). Fluorescence-activated cell sorting acquisition and sorting were performed on LSR-Fortessa (BD) and Aria III (BD), respectively. Analysis was performed using the FlowJo software (Tree star). In vitro culture To address the regulation of GM-CSF, sorted naive T H cells were stimulated for 5 days with 1 μg ml −1 anti-human CD3 (OKT3, Bioexcel) antibody with or without 1 μg ml −1 anti-human CD28 (CD28.2, BD Pharmingen) and 10 ng ml −1 of one of the following cytokines: IL-1β, IL-6, IL-23, IL-2, IL-4, IL-7, IL-9, IL-15, IL-21 and TGF-β1 (all from PeproTech). Proliferation was assessed by labelling cells with 5 μM carboxyfluorescein succinimidyl ester (CFSE). Where indicated, 10 μg ml −1 of anti-human IL-2Rα (Basiliximab, Novartis) was added to the culture on day 0. To simultaneously analyse GM-CSF production and STAT5 phosphorylation, T H cells were cultured as described above. For inhibition of STAT5 phosphorylation, 2.5 μg ml −1 pimozide (Sigma) was added at day 0 and flow cytometric readouts were performed at day 5. For IL-2 restimulation of PBMCs obtained from healthy donors, CD4 + T cells were purified by magnetic-activated cell sorting separation (Miltenyi Biotech), as suggested by the supplier. IL-2 was added in concentrations ranging from 0 to 10 ng ml −1 and T H cells were cultured for 4 days at 37 °C. The impact of T reg cells on GM-CSF production was determined by co-culture of sorted naive (labelled with CFSE, eBiosciences) and regulatory T H cells (labelled with CellTrace Violet, Lifetechnologies) at a 1:1 ratio for 5 days. The cells were stimulated with and anti-CD3 plus anti-CD28 antibodies. Where indicated, 10 μg ml −1 anti-TGF-β and anti-IL-10R (Biolegend) were added to the co-culture at day 0. STAT5 phosphorylation PBMCs, sorted naive T H cells or naive T H cells together with T reg cells were stimulated for 10 min at 37 °C with 10 ng ml −1 of the indicated cytokine. Cells were then fixed in 1.6% paraformaldehyde and permeabilzed in methanol on ice for 30 min. PBMC isolation, cryopreservation and thawing PBMCs were isolated by density gradient centrifugation using Lympholyte-H (Cedarlanes). PBMCs were cryopreserved in sterile-filtered fetal calf serum (Biochrom)+10% dimethyl sulfoxide (Applichem) at a final concentration of 2.5 × 10 6 ml −1 and stored in liquid nitrogen. Cyrovials were thawed in a 37 °C water bath and washed twice by drop-wise addition of 37 °C RPMI-1640 (PAN biotech) with 10% fetal calf serum. Microscopy Sorted naive T H cells (CFSE labelled) and T reg cells (CellTrace Violet labelled) were placed on cover slide, pretreated with poly-l-lysine and allowed to rest for 30 min. IL-2Fc (Sigma) (10 ng ml −1 ) was added for 10 min before cells were washed and fixed with 1:1 aceton:methanol for 12 h at −20 °C. IL-2Fc was then stained with APC-conjugated anti-human IgG antibodies (G18–145, BD Biosciences). Fluorescent imaging was performed using an inverted fluorescent microscope with a × 40 objective (IX81, Olympus). Enzyme-linked immunosorbent assay Cytokine levels of cell culture supernatants and human serum were analysed by enzyme-linked immunosorbent assay as suggested by the supplier (all Mabtech). CSF levels of MMP9 and NFL were determined as previously described [36] . Quantitative real-time PCR RNA was isolated with the PureLink RNA Micro Kit and complementary DNA was obtained using SuperScript III reverse transcriptase (both Life Technologies). Quantitative PCR was then performed using the CSF2 and GAPDH TaqMan gene expression assay (Life Technologies) and read on a CFX384 Touch Real-Time PCR Detection System (Bio-Rad). Statistical analysis All statistical tests were performed using the R statistical software package or Prism 5 (GraphPad). Differences between two groups were analysed using a two-sided t -test, accounting for different variances by Welch’s correction if indicated. Non-gaussian distributions were compared by the nonparametric Mann–Whitney test. Analysis of variance was used to compare >2 groups and regression analysis was used to test for correlations between genotype and flow cytometric data, controlling for age and sex. Gene-dosage effects were analysed by linear regression, assuming a linear genotype–phenotype correlation. We estimated the sample size considering the variation and mean of the distribution. How to cite this article: Hartmann, F. J. et al . Multiple sclerosis-associated IL2RA polymorphism controls GM-CSF production in human T H cells. Nat. Commun. 5:5056 doi: 10.1038/ncomms6056 (2014).